Regulation of A20 and other OTU deubiquitinases by reversible oxidation Protein ubiquitination is a highly versatile post-translational modification that regulates as diverse processes as protein degradation and kinase activation. Deubiquitinases hydrolyse ubiquitin modifications from proteins and are hence key regulators of the ubiquitin system. Ovarian tumour deubiquitinases comprise a family of fourteen human enzymes, many of which regulate cellular signalling pathways. Ovarian tumour deubiquitinases are cysteine proteases that cleave polyubiquitin chains in vitro and in cells, but little is currently known about their regulation. Here we show that ovarian tumour deubiquitinases are susceptible to reversible oxidation of the catalytic cysteine residue. High-resolution crystal structures of the catalytic domain of A20 in four different oxidation states reveal that the reversible form of A20 oxidation is a cysteine sulphenic acid intermediate, which is stabilised by the architecture of the catalytic centre. Using chemical tools to detect sulphenic acid intermediates, we show that many ovarian tumour deubiquitinases undergo reversible oxidation upon treatment with H 2 O 2 , revealing a new mechanism to regulate deubiquitinase activity. Protein ubiquitination is a key regulatory mechanism in which the small protein ubiquitin (Ub) is covalently attached to, most commonly, Lys residues of proteins [1] . Ubiquitination on substrates can comprise a single molecule (monoubiquitination) or a Ub chain (polyubiquitination). Polyubiquitin (polyUb) signals differ in structure and function depending on the linkage type within the polyUb chain. Indeed, the eight distinct Ub chain linkages coexist in cells, and appear to have distinct functions [2] , [3] . While Lys48- and Lys11-linked Ub polymers target proteins for proteasomal degradation, Lys63- and Met1-linked polyUb regulate non-degradative functions such as activation of protein kinase cascades during NF-κB (nuclear factor-κB) activation [2] , [3] . Ub modifications are reversed by five families of altogether ~80 active deubiquitinases (DUBs) in human cells, and many of these DUBs are emerging as important regulators of the Ub system [4] , [5] . For example, several DUBs have been described to regulate the transcription factor NF-κB (ref. 6 ), activation of which depends on an intricate network of both degradative and non-degradative Ub signals [3] , [7] . The best-studied DUB in this pathway is the ovarian tumour (OTU) enzyme A20 (refs 8 , 9 ). A20 is a tumour suppressor, and its deletion in mice results in hyperinflammatory phenotypes consistent with deregulated NF-κB signalling. Mechanistically, A20 establishes a powerful negative feedback loop [8] , [9] . A20 is thought to perform its functions by ‘editing’ Ub chains, that is, by replacing non-degradative Lys63-linked Ub chains with degradative Lys48-linked Ub chains on key ubiquitination substrates (for example, RIP1) in the NF-κB activation cascade [10] , [11] . This editing capability is facilitated by an N-terminal OTU DUB domain to hydrolyse Ub chains, and by seven C-terminal ZnF domains that bind Ub and, either directly or indirectly, act as an E3-ligase [9] , [10] . Inflammation arising as result of A20 deficiency exemplifies that Ub chain assembly and disassembly have to be carefully regulated to generate an appropriate signal. However, mechanisms of DUB inhibition that could amplify Ub signalling have remained elusive. To elucidate such global mechanisms of enzyme regulation, much can be learned from similar reversible post-translational modification systems, such as protein phosphorylation. Protein phosphatases antagonize the activity of protein kinases, and several mechanisms regulating their activity have been reported; one such mechanism is their regulation by reversible oxidation [12] . Many phosphatases are reversibly inactivated by reactive oxygen species (ROS) such as H 2 O 2 , a second messenger that is rapidly produced in cells in response to stimuli such as cytokines, growth factors and DNA damage, leading to increased phosphorylation of cellular proteins [13] , [14] , [15] , [16] , [17] . Mechanistic and structural studies have shown that ROS predominantly target Cys residues in proteins, in particular low pK a Cys residues that are commonly found in the active site of enzymes. Such Cys residues can be first oxidized to a sulphenic acid intermediate (SOH, ‘sulphenylated’), which is reversible by reducing agents [13] . Sulphenylated Cys residues undergo further oxidation to sulphinic (SO 2 H) or sulphonic (SO 3 H) acid and these higher oxidation states are irreversible. Other forms of reversible Cys oxidation are the formation of a disulphide bridge between two nearby Cys residues [18] , or the formation of a cyclic sulphenamide, as a result of a covalent bond formed between the Cys and the main chain nitrogen of a neighbouring residue [19] , [20] . These two latter mechanisms prevent overoxidation of susceptible Cys residues to irreversible oxidation states. As four of the five known DUB classes are Cys proteases that contain low pK a Cys residues in their active site, we asked whether DUBs are reversibly regulated by ROS. We found that A20 and other OTU enzymes undergo sulphenylation of their catalytic Cys residue in the presence of low concentrations of H 2 O 2 . High-resolution crystal structures of the A20 OTU domain in different oxidation states reveal how the usually unstable SOH intermediate is stabilised by the architecture of the OTU catalytic centre, in a mechanism that may be shared by many OTU DUBs. Our findings reveal a new universal mechanism of DUB inhibition that may impact on the levels of ubiquitination in oxidative stress conditions. Reducing agents activate the A20 DUB Previous characterization of A20 DUB activity and linkage-specificity using in vitro DUB assays has shown that it cleaves Lys48-linked chains. We performed DUB assays with the catalytic domain of A20 (ref. 21 ) against three chain types. Purified A20 that had been freeze-thawed showed weak activity towards diUb, in the absence of reducing agents in the reaction ( Fig. 1a ). Preincubation of A20 with 10 mM dithiothreitol (DTT) before the reaction increased A20 DUB activity against Lys48-linked chains, but not Lys63- or Met1-linked chains consistent with previous studies [22] . We further tested the effects of reducing agents on A20 activity by incubating the DUB with increasing amounts of DTT for 15 min, and assaying its activity against Lys48-linked triUb ( Fig. 1b ). While untreated A20 had weak activity, incubation of A20 with DTT increased the activity of the DUB significantly. DTT treatment had no effect on the proteins oligomeric state, as inactive freeze-thawed A20 was still monomeric, monodisperse and readily crystallized (see below). 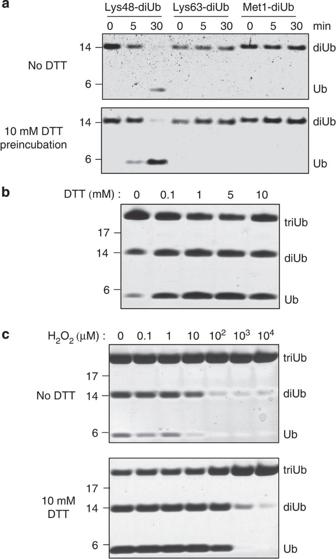Figure 1: Reversible A20 oxidationin vitro. (a) DUB assay of A20 OTU against Lys48-, Lys63- and Met1-linked diUb. The DUB assay was carried out either in the absence of reducing agents in the reaction buffer (upper panel) or the DUB was first preincubated with 10 mM DTT for 15 min before the DUB assay. (b) DUB assay of A20 OTU against Lys48-linked triUb was performed with preincubation of the OTU in increasing concentrations of DTT. The reaction was carried out in buffer lacking DTT. (c) A20 was first incubated with indicated concentrations of H2O2for 15 min at 23°C, and 100 U of catalase was added to quench the H2O2. To one half of the sample, DTT was added to a final concentration of 10 mM and incubated at room temperature for 15 min. The activity of the treated A20 was tested in a DUB assay using Lys48-linked triUb as substrate. Figure 1: Reversible A20 oxidation in vitro . ( a ) DUB assay of A20 OTU against Lys48-, Lys63- and Met1-linked diUb. The DUB assay was carried out either in the absence of reducing agents in the reaction buffer (upper panel) or the DUB was first preincubated with 10 mM DTT for 15 min before the DUB assay. ( b ) DUB assay of A20 OTU against Lys48-linked triUb was performed with preincubation of the OTU in increasing concentrations of DTT. The reaction was carried out in buffer lacking DTT. ( c ) A20 was first incubated with indicated concentrations of H 2 O 2 for 15 min at 23°C, and 100 U of catalase was added to quench the H 2 O 2 . To one half of the sample, DTT was added to a final concentration of 10 mM and incubated at room temperature for 15 min. The activity of the treated A20 was tested in a DUB assay using Lys48-linked triUb as substrate. Full size image The effect of reducing agents on A20 activity suggested that the enzyme is susceptible to regulation by ROS. To test this hypothesis, we first treated 5 μM A20 with increasing amounts of H 2 O 2 in vitro for 15 min. Catalase was added to rapidly deplete H 2 O 2 , and stop oxidation. Samples were then split and to one half, 10 mM DTT was added and incubated for 15 min at room temperature. The proteins were used in DUB assays against Lys48-linked triUb ( Fig. 1c ). This experiment revealed that H 2 O 2 concentrations exceeding 10 μM significantly reduced A20 DUB activity. Importantly, this inhibition was completely reversed by DTT up to a H 2 O 2 concentration of 100 μM, suggesting fully reversible inhibition of A20 DUB activity in the physiologically important range of 10–100 μM H 2 O 2 . Incubation with higher concentrations of H 2 O 2 (1 mM) led to irreversible inhibition that could not be reversed by subsequent DTT treatment. Overall, these results indicated that ROS-mediated oxidation of A20 can be reversed by DTT treatment, allowing for reversible regulation of enzyme activity. Our previous A20 structure suggested that the active site of A20 is catalytically competent [21] , generating a low pK a Cys103 as the most likely target of oxidation. However, the mechanism of reversible oxidation, and the involvement of the remaining six further Cys residues present in the analysed A20 OTU domain construct (amino acids 1–366, ( [21] )) was unclear ( Fig. 2a ). 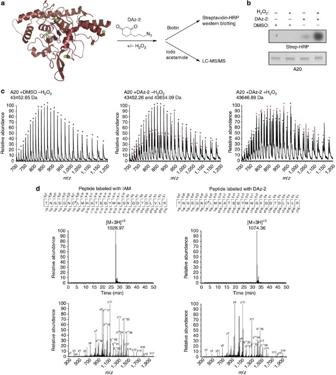Figure 2: Detection of SOH in reversibly oxidized A20. (a) Schematic of the reaction. Structure of A20 (pdb-id 2vfj (21)) showing the six ordered Cys residues (green). Treatment of A20 with dimedone derivatives, such as DAz-2, tests for Cys SOH intermediates, which can be detected by western blotting (as inb) or by mass-spectrometry (as inc) (b) Purified A20 was treated with 50 μM H2O2for 60 min at room temperature and incubated with dimethylsulphoxide or DAz-2. Subsequent biotinylation allows detection of A20 modification by Strepavidin-coupled horseradish peroxidase (Strep-horseradish peroxidase (HRP)). (c)Left,mass-spectra of intact A20 OTU domain (calculated mass 43452 Da, labelled with black asterisks) without H2O2treatment.Middle, untreated A20 OTU domain labelled with DAz-2.Right, A20 OTU domain treated with 50 μM H2O2for 1 h at room temperature, and labelled with DAz-2. Labelling with DAz-2 (195 Da) results in a second peak (labelled with red asterisks) in untreated and H2O2treated samples (observed mass 43654/43646, respectively). The observed mass corresponds to A20 labelled with one molecule of DAz-2. (d) Tryptic analysis of unlabelled (left) and labelled (right) A20 reveals the Cys103-containing peptide to be modified with DAz-2 (seeMethods). Shown is the sequence of the Cys103 containing tryptic peptide including b- and y-ions (top), extracted ion chromatograms (middle), and MS/MS spectra after collision-induced dissociation (bottom). The MS/MS spectra after collision-induced dissociation of precursor ion 1074.36 [M+3H]+3yielded specific b and y ions pertaining to the peptide with DAz-2 modification at Cys103. Figure 2: Detection of SOH in reversibly oxidized A20. ( a ) Schematic of the reaction. Structure of A20 (pdb-id 2vfj ( [21] )) showing the six ordered Cys residues (green). Treatment of A20 with dimedone derivatives, such as DAz-2, tests for Cys SOH intermediates, which can be detected by western blotting (as in b ) or by mass-spectrometry (as in c ) ( b ) Purified A20 was treated with 50 μM H 2 O 2 for 60 min at room temperature and incubated with dimethylsulphoxide or DAz-2. Subsequent biotinylation allows detection of A20 modification by Strepavidin-coupled horseradish peroxidase (Strep-horseradish peroxidase (HRP)). ( c ) Left, mass-spectra of intact A20 OTU domain (calculated mass 43452 Da, labelled with black asterisks) without H 2 O 2 treatment. Middle , untreated A20 OTU domain labelled with DAz-2. Right , A20 OTU domain treated with 50 μM H 2 O 2 for 1 h at room temperature, and labelled with DAz-2. Labelling with DAz-2 (195 Da) results in a second peak (labelled with red asterisks) in untreated and H 2 O 2 treated samples (observed mass 43654/43646, respectively). The observed mass corresponds to A20 labelled with one molecule of DAz-2. ( d ) Tryptic analysis of unlabelled (left) and labelled (right) A20 reveals the Cys103-containing peptide to be modified with DAz-2 (see Methods ). Shown is the sequence of the Cys103 containing tryptic peptide including b- and y-ions (top), extracted ion chromatograms (middle), and MS/MS spectra after collision-induced dissociation (bottom). The MS/MS spectra after collision-induced dissociation of precursor ion 1074.36 [M+3H] +3 yielded specific b and y ions pertaining to the peptide with DAz-2 modification at Cys103. Full size image Identification of an A20 SOH intermediate at Cys103 Recent advances in chemical biology allow for the direct detection of Cys SOH intermediates in proteins ( Fig. 2a ). Dimedone derivatives label hydroxylated thiol groups site-specifically, and can be used in conjunction with click-chemistry to append a reporter tag for the detection of sulphenylated proteins for further analysis by western blotting and/or mass-spectrometry [23] , [24] . To test whether A20 forms SOH intermediates, purified A20 OTU domain was incubated with either dimethylsulphoxide (control) or DAz-2 ( [24] ) during H 2 O 2 treatment in vitro . Subsequently, excess probe was removed and DAz-2 tagged proteins were conjugated to a biotin tag. DAz-2 treated A20 could be readily detected by western blotting before H 2 O 2 incubation, and labelling was significantly enhanced in the presence of H 2 O 2 ( Fig. 2b ), showing that A20 was indeed sulphenylated. To identify the site(s) of modification, A20 was subjected to mass-spectrometry analysis. The average intact mass of A20 was within 1 Da of the expected mass of unmodified A20 ( Fig. 2c ). Incubation with DAz-2 generated a second A20 species with lower abundance in the untreated sample and a highly abundant species with a mass-increase of 194 Da in the H 2 O 2 treated sample. The higher mass corresponds to A20 labelled with one molecule of DAz-2 (MW 195.2 Da) ( Fig. 2c ). Mass-spectrometry (MS)/MS analysis was used to identify the site of A20 modification by DAz-2. For this, samples were treated with iodoacetamide (IAM) to block unwanted reactions of free Cys residues, and then digested by trypsin. A triply charged precursor ion derived from the tryptic peptide containing the catalytic Cys103 was identified to be IAM labelled in untreated sample, and DAz-2-labelled in the H 2 O 2 treated reaction ( Fig. 2d ). This revealed that the catalytic Cys103 of A20 undergoes modification to SOH in the presence of H 2 O 2 , likely explaining the observed inhibition of enzyme activity by ROS. Molecular basis for A20 inhibition by reversible oxidation Having identified sulphenylation of A20 at Cys103, we set out to understand how this Cys modification was stabilised within the A20 catalytic site. We used X-ray crystallography to understand A20 regulation by ROS at the molecular level. High-resolution crystal structures are required to resolve oxidation of Cys residues. Published A20 OTU domain structures are either of too low resolution (3.2 Å, ( [21] )) or suffer from crystal twinning (2.5 Å, ( [25] )). We obtained a new high-resolution (<2.0 Å) crystal form for the A20 OTU domain ( Fig. 3a ), and performed oxidation studies on these crystals (see Methods ), to analyse the oxidation states of the catalytic Cys. 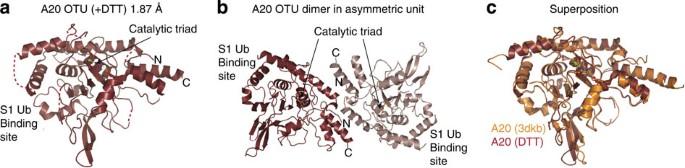Figure 3: A high-resolution crystal form for A20 OTU. (a) Structure of A20 OTU domain (amino acids (aa) 1–366) inP1 space group at 1.87 Å resolution. N- and C-terminus and the presumed S1 Ub binding site (from analogy with other OTU complexes, for example,40) are indicated. Residues of the catalytic triad (Cys103, His256, Asp70) are shown. Dotted lines indicate connectivity of disordered surface loops. (b) Structure of the A20 OTU dimer in the asymmetric unit. (c) Superposition of A20 OTU from this study (red) and from a previous study (pdb-id 3dkb, (25)). RMSD between structures is 0.8 Å over 322/352 residues. Figure 3: A high-resolution crystal form for A20 OTU. ( a ) Structure of A20 OTU domain (amino acids (aa) 1–366) in P 1 space group at 1.87 Å resolution. N- and C-terminus and the presumed S1 Ub binding site (from analogy with other OTU complexes, for example, [40] ) are indicated. Residues of the catalytic triad (Cys103, His256, Asp70) are shown. Dotted lines indicate connectivity of disordered surface loops. ( b ) Structure of the A20 OTU dimer in the asymmetric unit. ( c ) Superposition of A20 OTU from this study (red) and from a previous study (pdb-id 3dkb, ( [25] )). RMSD between structures is 0.8 Å over 322/352 residues. Full size image Crystals were grown in the presence or absence of DTT in mother liquor and protein to generate a reduced, active structure of A20, as well as a reversibly oxidized structure of A20, respectively. Some crystals grown in the absence of DTT were further treated with 50 μM H 2 O 2 for 60 or 270 min in soaking experiments. Data were collected to high resolution (1.84–2.20 Å, Table 1 ) at the Diamond Light Source, beamline I-02. Crystals belonged to space group P 1 with two A20 molecules in the asymmetric unit ( Fig. 3b ). Structures were determined by molecular replacement using the previously published A20 structure as a search model, and refined to final statistics shown in Table 1 . Table 1 Data collection and refinement statistics. Full size table The high-resolution structure of A20 OTU is almost identical to previously determined structures, with root-mean-square deviation (RMSD) values of <0.8 Å ( Fig. 3c ). There are no large-scale conformational changes, and most loops absent in the previous structures are also disordered in the new crystal form ( Fig. 3a ). The catalytic centre of the A20 OTU domain is in an identical conformation in which the catalytic His residue deprotonates the thiol group of the catalytic Cys103, increasing its reactivity ( Fig. 4a ). 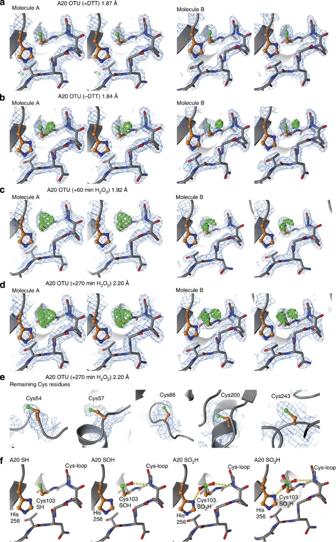Figure 4: The A20 catalytic triad in different oxidation states. (a–d) Stereo images of the catalytic Cys and His residues and the Cys-loop in A20. A 2|Fo|-|Fc| map (blue) contoured at 1.5 σ, and a |Fo|-|Fc| map (green, thick lines) contoured at 3.5 σ covers shown residues.Left:Molecule A of the asymmetric unit.Right:Molecule B of the asymmetric unit. (a) Structure of A20 in reduced, active state, grown in the presence of DTT. (b) Structure of A20 with reversible oxidized Cys103 SOH, from untreated crystals. (c) Structure of A20 with irreversibly oxidized Cys103 after incubation with 50 μM H2O2for 60 min. Cys residues were modelled as sulphinic and sulphonic acid in the two molecules, respectively. (d) Structure of A20 after 270 min incubation with 50 μM H2O2, modelled as inc. (e) The remaining ordered Cys residues in A20 (Cys54, Cys57, Cys86, Cys200, Cys243) are unaffected even after soaking for 270 min in 50 μM H2O2. Individual Cys residues are shown with 2|Fo|-|Fc| map (blue, contoured at 1.5 σ) and |Fo|-|Fc| map (green, contoured at 3.5 σ). There is no unmodelled density at these sites. (f) Final, refined models for reduced (A20 SH), reversibly oxidized (A20 SOH) and irreversibly (A20 SO2H, A20 SO3H) oxidized forms of A20. Yellow dotted lines indicate hydrogen bonds formed by oxidized Cys103. Figure 4: The A20 catalytic triad in different oxidation states. ( a – d ) Stereo images of the catalytic Cys and His residues and the Cys-loop in A20. A 2|F o |-|F c | map (blue) contoured at 1.5 σ, and a |F o |-|F c | map (green, thick lines) contoured at 3.5 σ covers shown residues. Left: Molecule A of the asymmetric unit. Right: Molecule B of the asymmetric unit. ( a ) Structure of A20 in reduced, active state, grown in the presence of DTT. ( b ) Structure of A20 with reversible oxidized Cys103 SOH, from untreated crystals. ( c ) Structure of A20 with irreversibly oxidized Cys103 after incubation with 50 μM H 2 O 2 for 60 min. Cys residues were modelled as sulphinic and sulphonic acid in the two molecules, respectively. ( d ) Structure of A20 after 270 min incubation with 50 μM H 2 O 2 , modelled as in c . ( e ) The remaining ordered Cys residues in A20 (Cys54, Cys57, Cys86, Cys200, Cys243) are unaffected even after soaking for 270 min in 50 μM H 2 O 2 . Individual Cys residues are shown with 2|F o |-|F c | map (blue, contoured at 1.5 σ) and |F o |-|F c | map (green, contoured at 3.5 σ). There is no unmodelled density at these sites. ( f ) Final, refined models for reduced (A20 SH), reversibly oxidized (A20 SOH) and irreversibly (A20 SO 2 H, A20 SO 3 H) oxidized forms of A20. Yellow dotted lines indicate hydrogen bonds formed by oxidized Cys103. Full size image Cys103 is unambiguously defined in crystals grown in the presence of DTT ( Fig. 4a ). Importantly, in the absence of DTT, Cys103 shows additional positive |F o |-|F c | electron density at its thiol function in both molecules of the asymmetric unit ( Fig. 4b ). This additional electron density cannot be explained by alternate side-chain conformations, is too close for a water molecule, and represents Cys SOH (A20 SOH), the reversibly oxidized form of A20 ( Fig. 4b ). When these crystals were incubated in 50 μM H 2 O 2 for 60 or 270 min, further oxidation occurred that was modelled as either Cys sulphinic acid (A20 SO 2 H) or Cys sulphonic acid (A20 SO 3 H) ( Fig. 4c ). Cys103 was the only Cys affected by oxidation as the remaining five ordered Cys thiolate groups were clearly defined in electron density even after long H 2 O 2 incubations ( Fig. 4e ). Modelling of the different oxidation states of Cys103 in the final refined structures reveal that Cys SOH forms an additional backbone hydrogen with the loop preceding the catalytic Cys (Cys-loop) ( Fig. 4f ). Irreversibly oxidized states of A20 additionally form a second hydrogen bond with the catalytic His256 residue ( Fig. 4f ). The refined A20 SOH structure revealed the molecular basis for A20’s ability to be regulated by reversible oxidation, as the SOH intermediate of Cys103 is stabilised by the architecture of the OTU catalytic centre via hydrogen bond formation with the Cys-loop. This likely decreases the reactivity of Cys103 and stabilises Cys103 against further oxidation, which occurs only after prolonged H 2 O 2 treatment ( Fig. 4 ) or at high H 2 O 2 concentration ( Fig. 1c ). Cys SOH is common in OTU DUBs Stabilization of SOH by the catalytic architecture of A20 suggested that other OTU DUBs might be regulated in a similar manner. The 14 human OTU DUBs can be subclassified into three different groups based on the size of the catalytic domain [5] , but available structures show that the catalytic site and the position of the Cys-loop are highly conserved [5] . To test whether A20-like and other OTU DUBs are sulphenylated, we used a newly developed chemoselective probe, DYn-2, which labels sulphenylated proteins and harbours an alkyne handle for enhanced bioorthogonal ligation [26] ( Fig. 5a ). Purified OTU DUBs were incubated with increasing concentrations of H 2 O 2 for 15 min, and SOH modifications were detected by western blotting. A20 was modified by DYn-2 to a similar extent as compared with DAz-2 ( Fig. 5b ). Cezanne/OTUD7B is highly similar to A20, and was found to be sulphenylated at low μM H 2 O 2 concentrations. Higher concentrations (100 μM) abrogated the DYn-2 signal, perhaps indicating rapid irreversible oxidation ( Fig. 5c ). Importantly, sulphenylation of Cezanne is not observed when the catalytic Cys194 is mutated to Ala ( Fig. 5d ), indicating that also this enzyme is exclusively modified at its active site Cys. 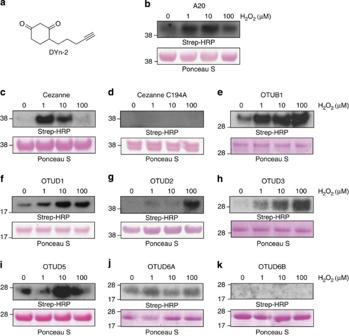Figure 5: Detection of sulphenylation in different OTU DUBs. (a) Chemical structure of DYn-2, which features an alkyne group. (b–k) Different human OTU family members were treated with increasing concentrations of H2O2for 15 min at room temperature. H2O2was quenched by adding 200 U catalase and the OTU was labelled with 1 μM DYn-2, which was subsequently biotinylated. The labelled proteins were detected by streptavidin-horseradish peroxidase (Strep-horseradish peroxidase (HRP)) western blot. Ponceau S staining of the membrane confirmed equal loading of proteins. (b) A20 OTU domain (aa 1–366), (c) Cezanne/OTUD7b (aa 124–438), (d) Cezanne/OTUD7b C194A (aa 124–438), (e) OTUB1 (aa 1–271, full length), (f) OTUD1 (aa 287–481), (g) OTUD2 (aa 1–348, full length), (h) OTUD3 (aa 52–275), (i) OTUD5/DUBA (aa 171–358), (j) OTUD6A (aa 128–288), (k) OTUD6B (aa 133–293). Figure 5: Detection of sulphenylation in different OTU DUBs. ( a ) Chemical structure of DYn-2, which features an alkyne group. ( b–k ) Different human OTU family members were treated with increasing concentrations of H 2 O 2 for 15 min at room temperature. H 2 O 2 was quenched by adding 200 U catalase and the OTU was labelled with 1 μM DYn-2, which was subsequently biotinylated. The labelled proteins were detected by streptavidin-horseradish peroxidase (Strep-horseradish peroxidase (HRP)) western blot. Ponceau S staining of the membrane confirmed equal loading of proteins. ( b ) A20 OTU domain (aa 1–366), ( c ) Cezanne/OTUD7b (aa 124–438), ( d ) Cezanne/OTUD7b C194A (aa 124–438), ( e ) OTUB1 (aa 1–271, full length), ( f ) OTUD1 (aa 287–481), ( g ) OTUD2 (aa 1–348, full length), ( h ) OTUD3 (aa 52–275), ( i ) OTUD5/DUBA (aa 171–358), ( j ) OTUD6A (aa 128–288), ( k ) OTUD6B (aa 133–293). Full size image Furthermore, sulphenylation was also detected in OTUB1, OTUD1, OTUD2, OTUD3, OTUD5 and OTUD6A ( Fig. 5e–j ) but not in OTUD6B ( Fig. 5k ). DYn-2 modification was observed in untreated samples of OTUB1, OTUD1, OTUD5 and OTUD6A suggesting that a significant fraction of the purified enzyme is (reversibly) oxidized. OTUD1, OTUD3 and OTUD5 show a similar profile as compared to A20 ( Fig. 5 ), while OTUD2 is sulphenylated only at the highest H 2 O 2 concentration ( Fig. 5g ). Collectively, these results show that OTU family DUBs are readily sulphenylated in response to ROS. Furthermore, the observed differences in modification suggest that ROS may gradually regulate DUB activity. Generation of ROS in cells constitutes an important signalling event, however its transient nature, high reactivity and high diffusion rate pose challenges for detecting the roles and targets of ROS. To date, protein tyrosine phosphatases are the best-studied enzyme class regulated by ROS, and the impact of ROS production in phosphorylation cascades is unquestioned. Phosphatases were also instrumental to illuminate the different mechanisms of reversible inhibition of enzyme activity by oxidation [27] . The arrival of new tools to detect modified forms of proteins, such as dimedone derivatives that label SOH [24] or antibodies against cyclic sulphenamides [28] have confirmed many targets of ROS in cells, and have opened new avenues to study the global effects of oxidative stress. Moreover, the application of these tools to proteomics has led to the identification of many new Cys-modified proteins including kinases, peroxidases and DUBs [24] , [29] . We report that OTU DUBs can be regulated by reversible oxidation of the catalytic Cys, and provide structural and biochemical evidence that this is mediated by a Cys SOH intermediate, which is particularly suitable to be stabilised by the architecture of the OTU active site, in which conserved residues in the loop preceding the catalytic Cys residue (Cys-loop) stabilize the added hydroxyl group. Oxidation of DUBs is perhaps not surprising as most are Cys proteases, but what could be significant is the reversibility and the varying sensitivity of OTU DUBs to H 2 O 2 concentrations, as this suggests that some DUBs (for example, Cezanne) are remarkably sensitive to H 2 O 2 , while others (for example, OTUD2) are not. This difference in sensitivity could arise from the architecture of the catalytic centre. Moreover, it is tempting to speculate that inactive conformations observed for some DUBs in the absence of Ub substrate [4] may represent a protective mechanism, where the DUB only forms a reactive catalytic Cys in the presence of its substrate or an activating interaction partner. Reversible oxidation of Cys proteases has been studied in, for example, Cys Cathepsins [30] , but was unknown for DUBs. While this manuscript was under review, Cotto-Rios et al . [31] reported reversible oxidation via SOH intermediates for several USP family members and for UCH-L1, DUBs which are structurally unrelated to OTU DUBs. The authors could show that USP1 was reversibly inactivated in cells in response to oxidative DNA damage, leading to increased PCNA ubiquitination, suggesting in vivo relevance for this new regulatory mechanism. Reversible oxidation has further been studied for small Ub-like modifier (SUMO) proteases of the Sentrin/SUMO-specific protease (SENP) family, and while these enzymes were shown to undergo reversible crosslinking as well as sulphenylation [32] , the required concentrations of H 2 O 2 were significantly higher (4–10 mM) as compared with OTU DUBs [32] . In addition, ROS also regulate the activity of Atg4, a Sentrin/SUMO-specific protease-fold protease responsible for hydrolysis of Atg8, during autophagy [33] . Most enzymes in the Ub system utilize catalytic Cys residues. E1 Ub activating enzymes, E2 Ub conjugating enzymes and subclasses of E3 Ub ligases transfer Ub via thioester intermediates [2] , [3] . Little is known whether oxidative stress can regulate assembly of Ub conjugates. This has however been studied for the SUMO cascade enzymes. An elegant paper showed that H 2 O 2 treatment of cells leads to decrease of SUMO conjugates by crosslinking SUMO E1 with Ubc9, the SUMO E2 via reversible disulphide bridges [34] . Together, these data highlight that the enzymes in ubiquitination and Ub-like modification, and in particular the proteases in these systems are new targets of ROS in cells. The next challenge will be to define cellular situations in which OTU oxidation occurs. A role for H 2 O 2 in augmenting NF-κB signalling has been suggested by many studies. Interestingly, combined treatment of cells with tumour-necrosis factor-α and H 2 O 2 leads to prolonged changes in the kinetics of NF-κB nuclear translocation, and sustained polyubiquitination of RIP1, suggesting that DUBs may be affected [35] . While the authors implicated Cezanne in this process, it could also be A20 that mediates the reported effects. Elevated levels of ROS have been found in many disease states, notably cancer, diabetes and conditions of chronic inflammation [36] . Given the role of deregulation of ubiquitination in disease pathogenesis [37] , it is possible that oxidative stress exerts its pathological functions, at least in part, also via deregulation of DUBs. The realization that DUBs are a target of ROS may lead to re-evaluation of cell signalling processes in oxidative stress-induced conditions. DUB purification A20 (residues 1–366) was purified as a GST fusion protein as described previously [21] . In short, protein is expressed in E. coli BL21 or Rosetta2 cells, lysed in lysis buffer (270 mM sucrose, 50 mM Tris (pH 8.0), 1 mM EDTA, 50 mM sodium fluoride, 10 mM 2-mercaptoethanol, 0.1 mg ml −1 DNaseI, 1 mg ml −1 lysozyme, Complete protease inhibitor (Roche)) and affinity purified by Glutathione S-Sepharose 4B (GE Healthcare). Cleavage of the tag by PreScission protease was followed by anion exchange (HiTrap Q FF) and gel filtration in buffer 1 (200 mM NaCl, 25 mM Tris (pH 8.5), 5 mM DTT), resulting in pure protein. The A20 protein used for crystallization contained a single point mutation G114S remote from the active site that does not alter the structure. Other OTU DUBs described in this study were expressed as GST fusion proteins in bacteria and purified as above. Deubiquitinase assays DUB assays were performed according to [22] . DUBs were diluted to 2 × final concentration in 150 mM NaCl, 25 mM Tris (pH 7.5) and 10 mM DTT and used directly, or activated at 23 °C for 10 min. Subsequently, 10 μl of diluted enzyme were mixed with 1–2 μg diUb and 2 μl of 10 × DUB buffer (500 mM NaCl, 500 mM Tris (pH 7.5) and 50 mM DTT) in a 20 μl reaction. For oxidation studies, A20 was preactivated with 10 mM DTT, and subsequently dialysed against degassed reaction buffer lacking DTT. Protein was incubated with indicated concentrations of H 2 O 2 for 15 min, and either used in a DUB reaction, or again DTT-treated (10 mM, 15 min) and used in a DUB reaction. Reactions were incubated at 37 °C and 6 μl aliquots were taken at indicated times, and mixed with 4 μl lithium dodecyl sulfate (LDS) sample buffer containing 100 mM DTT to stop the reaction. Reactions were resolved on 4–12% NuPage SDS–polyacrylamide gel electrophoresis gradient gels run in MES buffer, and stained using the Silver Stain Plus kit (BioRad). Labelling of OTU DUBs with DAz-2 A20 was treated with 20 mM DTT for 10 min at room temperature. Excess DTT was removed with a P-6 micro BioSpin column (BioRad) that had been pre-equilibrated with 20 mM Tris-HCl pH 7.2, 150 mM NaCl. 25 μM A20 was labelled with 10 mM DAz-2 and treated with 50 μM H 2 O 2 for 1 h at room temperature while rocking. Protein was buffer exchanged into 25 mM ammonium bicarbonate pH 8.0, using an Amicon ultracentrifugal filter with a 10-kDa Molecular weight cut-off (MWCO) (Millipore). The DAz-2 labelled samples were concentrated to dryness via vacuum centrifugation, then resuspended in 50 mM triethanolamine pH 7.4 and 1% SDS. Probe modified proteins were detected via bioorthogonal Huisgen (3+2) cycloaddition by incubating with 100 μM YnBiotin, 1 mM Tris (2-carboxyethyl) phosphine hydrochloride (TCEP), 100 μM tris[(1-benzyl-1H-1,2,3-triazol- 4-yl)methyl]amine ligand (TBTA), and 1 mM CuSO 4 for 1 h at room temperature while rocking. The protein was methanol precipitated to remove excess reagents. Protein samples were resuspended in Laemmli buffer containing 10% (v/v) β-mercaptoethanol. The samples were separated by SDS–polyacrylamide gel electrophoresis using Mini-Protean TGX 4–15% Tris-Glycine gels (BioRad) and transferred to a polyvinylidene difluoride (PVDF) membrane (BioRad). After transfer, the PVDF membrane was blocked with 3% bovine serum albumin for 1 h at room temperature. The membrane was washed with Tris-buffered saline Tween-20 buffer (TBST) (2 × 10 min) and then incubated with 1:80,000 Strep-horseradish peroxidase (GE-Healthcare). The PVDF membrane was washed with Tris-buffered saline Tween-20 buffer (TBST) (2 × 10 min) and then developed with chemiluminesence (GE Healthcare ECL Plus Western Blot Detection System) and imaged by film. Equal loading was assessed by staining the PVDF membrane with 50% R-250 Coomassie blue (Boston BioProducts) in 50% MeOH for 10 min. Intact mass analysis of A20 OTU DAz-2 labelled and unlabelled protein samples were submitted for intact mass analysis using an electrospray linear ion trap mass spectrometer (LTQ-XL, Thermo Scientific) after separation on an Agilent Eclipse XDG-C8 2.1 mM × 15 mm trap with mobile phases A (0.1% formic acid in water) and B (0.1% formic acid in acetonitrile), which was used to trap, desalt and elute proteins onto a Varian 2.1 mm × 50 mm 5 μm PLRP-S C18 column with a gradient of 5 to 100% B in 14 min at a flow rate of 200 μl min −1 . Liquid-chromatography–MS/MS analysis of A20 DAz-2 labelled and unlabelled samples were prepped for in-solution trypsin digestion by diluting the samples in 6 M urea/100 mM Tris-OH pH 7.2. The protein was reduced with 10 mM DTT for 1 h at room temperature. The samples were subsequently alkylated with 55 mM IAM for 1 h at room temperature in the dark. Excess IAM was quenched with the addition of 55 mM DTT and allowed to react for 30 min at room temperature. The urea concentration was diluted to less than 2 M by addition of 25 mM ammonium bicarbonate pH 8.0. Sequencing grade trypsin (Promega) was added at a ratio of 1:25 (w/w) and incubated overnight at 37 °C. The sample was concentrated by vacuum centrifugation and desalted with a C18 column (Nest Group). Peptide samples were analysed on an electrospray linear ion trap mass spectrometer (LTQ-XL, Thermo Scientific) after separation on an Agilent Eclipse XDB-C8 2.1 mm × 15 mm trap with mobile phases A (0.1% formic acid in water) and B (0.1% formic acid in acetonitrile), which was used to trap, desalt, and elute the peptides onto a Vydac Everest reverse-phase C18 monomeric column (2.1 mm × 150 mm, 300 Å, 5 μm) with a gradient of 5 to 60% B in 60 min at a flow rate of 200 μl min −1 . Peptide and protein identification was done through the Mascot search programme ( http://www.matrixscience.com ). Mass lists, in the form of Mascot generic files, were created automatically and used as the input for Mascot MS/MS ion searches against a database containing the full sequence of A20. The search parameters were as follows. The enzyme specificity was Trypsin with one missed cleavage permitted. The variable modifications included Carbamidomethyl (C-SH), DAz-2 (C-SOH) and Oxidation (M). The mass tolerance for the precursor ions obtained from the ESI-Trap was set to±2 Da and the fragment mass tolerance was set to±0.8 Da. The maximum expectation value ( p ) for accepting individual MS/MS spectra was set at 0.05. A20 crystallization and structure determination Crystallization was performed in hanging drop set-up, and large crystals in P 1 space group formed at a protein concentration of 6–8 mg ml −1 from 2–2.5 M NaCl, 0.1 M MES (pH 6–6.7). Crystals grew after 4 days, and reached maximum size after 1–2 weeks. Untreated A20 crystals corresponded to reversibly oxidized Cys SOH form of A20 (A20 SOH). DTT (10 mM) was added to the crystallization mother liquor, protein solution and cryo-protectant solution to obtain the reduced active A20 structure (A20 SH). Soaks of crystals in mother liquor containing 50 μM fresh H 2 O 2 for 60 or 270 min resulted in Cys sulphinic acid (A20 SO 2 H) and Cys sulphonic acid (A20 SO 3 H) forms of A20. Before vitrification in a nitrogen cryo stream, crystals were soaked in mother liquor containing 20% ethylene glycol. Synchrotron data was collected at the Diamond Light Source, beamline I-02, at 100 K and at wavelengths of 0.97950 (A20 SH) and 0.92000 (A20 SOH, A20 SO 2 H, A20 SO 3 H). Crystals displayed the space group P 1 with two molecules of A20 in the asymmetric unit. Phases were obtained by molecular replacement in Phaser using the previous A20 structure (2vfj, ( [21] )) as a search model. Subsequent rounds of model building in Coot [38] and refinement in Phenix [39] (using simulated annealing) resulted in final statistics shown in Table 1 . Less than 0.5% of all residues were Ramachandran outliers, and these residues were located in flexible loop regions. Labelling and detection of OTU sulphenylation using DYn-2 Labelling and detection using DYn-2 probes was performed as described [26] . The different DUBs were first treated with Tris (2-carboxyethyl) phosphine (TCEP) and DTT to completely reduce Cys residues, and subsequently buffer exchanged using P-6 micro Biospin columns (BioRad) to remove reducing agents. OTU DUBs were treated with H 2 O 2 in the concentration range of 0–100 mM for 15 min at 23°C. Catalase was added to deplete H 2 O 2 and the proteins labelled with DYn-2. After labelling, excess probe was removed and DYn-2 labelled proteins were conjugated to biotin, which could be detected by western blotting with streptavidin-horseradish peroxidase. Ponceau S (Sigma Aldrich) staining was used to detect total protein levels. Accession codes : Coordinates and structure factors for the reduced and oxidized forms of A20 have been deposited in the Protein Data Bank under accession codes 3zjd (A20 SH), 3zje (A20 SOH), 3zjg (A20 SO 2 H) and 3zjf (A20 SO 3 H). How to cite this article: Kulathu, Y. et al . Regulation of A20 and other OTU deubiquitinases by reversible oxidation. Nat. Commun. 4:1569 doi: 10.1038/ncomms2567 (2013).